Discovery of optimal zeolites for challenging separations and chemical transformations using predictive materials modeling Zeolites play numerous important roles in modern petroleum refineries and have the potential to advance the production of fuels and chemical feedstocks from renewable resources. The performance of a zeolite as separation medium and catalyst depends on its framework structure. To date, 213 framework types have been synthesized and >330,000 thermodynamically accessible zeolite structures have been predicted. Hence, identification of optimal zeolites for a given application from the large pool of candidate structures is attractive for accelerating the pace of materials discovery. Here we identify, through a large-scale, multi-step computational screening process, promising zeolite structures for two energy-related applications: the purification of ethanol from fermentation broths and the hydroisomerization of alkanes with 18–30 carbon atoms encountered in petroleum refining. These results demonstrate that predictive modelling and data-driven science can now be applied to solve some of the most challenging separation problems involving highly non-ideal mixtures and highly articulated compounds. Crude oil remains the dominant source for transportation fuels and chemical feedstocks. Improving the efficiency of oil refining will help to extend the supply and reduce the cost of current petroleum products. In the 1950s, crystalline zeolites containing sub-2 nm internal pores emerged as shape/size-selective sorbents and catalysts, leading to dramatic improvements in numerous processes utilized by the petrochemical industry [1] . For example, zeolites are used to catalyse the transformation of linear long-chain alkanes to slightly branched alkanes of similar molecular weight, with the goal of reducing the pour point and increasing the viscosity index of lubricant oils [2] , [3] , [4] , [5] . Similar transformations are also desirable for diesel and other fuel oils, in which shorter alkanes are involved. These hydroisomerization reactions depend on a delicate balance between the degree of framework confinement and the size of alkane molecules. A suitable zeolite possesses a high affinity for linear alkanes but low affinity for branched isomers, so that the desired mono-branched products are not being cracked into smaller species [4] . Separating ethanol from its aqueous solution, a process essential for biofuel production, currently relies on energy-intensive distillation [6] . Nearly defect-free silicalite-1, an all-silica zeolite with the framework type MFI, has been proposed as an effective sorbent and membrane for this separation [7] , [8] . All-silica zeolites by themselves are very hydrophobic, but the adsorption of ethanol can promote water co-adsorption through hydrogen bond formation and lower the selectivity [8] , [9] . For this application, the desired zeolite possesses a pore/channel system that accommodates ethanol molecules but disfavours hydrogen bonding with water molecules. Experimental testing of all existing zeolites for a given application would be very time and labour intensive, sometimes even infeasible when a synthesis protocol for the material with the desired composition is not yet developed. In addition, the possible number of synthesizable zeolites is enormously large [10] , with some of the structures from the predicted crystallography open database (PCOD) possessing potentially much better characteristics. Selecting optimal candidate materials through predictive modelling is hence a very attractive proposition. Such screening studies have so far focused mostly on single-component adsorption of small, rigid, non-hydrogen-bonding molecules, such as short hydrocarbons [11] , [12] , [13] , [14] , [15] , carbon dioxide (refs 13 , 16 , 17 , 18 , 19 ) and hydrogen (refs 13 , 20 ). Many of them rely on extrapolation of single-component data [12] , [16] , [17] , [18] to obtain mixture properties, and others rely predominantly on geometric analysis [13] . Screening sorbents and catalysts for complex mixtures composed of large, articulated molecules, where advanced algorithms are required for sampling the distribution of thousands of conformers, or polar, hydrogen-bonding molecules, where an accurate description of electrostatics and the resulting mixture non-idealities are of paramount importance, has so far been an intractable problem. Enabled by a multi-step screening workflow, efficient sampling algorithms, accurate force fields and a two-level parallel execution hierarchy (see Methods section for a detailed description) utilizing up to 131,072 compute cores on Mira, a leadership-class supercomputer at Argonne National Laboratory, we perform high-throughput screening for two energy-related applications and identify zeolites with exceptional selectivities for ethanol purification from aqueous solution and the transformation of alkanes with 18–30 carbon atoms. Ethanol/water separation Sugar fermentation produces ethanol with solution-phase concentrations from w =5 to 15 wt% at temperatures between 298 and 323 K depending on the yeast/sugar combination [21] , [22] . The adsorption selectivity of ethanol over water generally decreases with solution-phase ethanol concentration and temperature, with the dependence on the latter relatively small over the above temperature range [9] . For separation processes based on equilibrium adsorption, it is the final concentration of the raffinate that determines the composition of the adsorbed phase (retentate). The raffinate concentration would become very low when the process target is to adsorb most of the ethanol in a single step. Hence, we carry out Monte Carlo simulations at a solution-phase concentration of w =0.12 wt% and T =323 K to screen all of the framework structures available from the Structure Commission of the International Zeolite Association, IZA-SC [23] . We use the product of ethanol selectivity, S EtOH (= r (1− w )/(1− r ) w , where r is the retentate concentration), and loading, Q EtOH , to rank the zeolite structures. This performance metric, P EtOH , is rather robust and effective in identifying the top structures at a given target w , in the sense that its ranked-order distribution exhibits an exponential decay for the highly ranked structures (see Supplementary Fig. 1 ) and, as a result, the ranks of the most promising structures are less likely to be affected by simulation uncertainties. It should be noted that this performance metric is not tied to a particular separation process (for example, liquid or vapour phase adsorption, pressure or temperature swing, membrane permeation, batch or continuous operation), but instead tries to identify zeolites that are potentially good targets for many different processes by focusing on the two quantities that are key factors in any separation process. At the ambitiously low raffinate concentration of w =0.12 wt%, none of the candidate structures can achieve the selectivity target, S target ≥18,000, that would be required for the retentate to exceed the ethanol/water azeotropic point ( r ≥95.6 wt%; that is, S target ≥0.956(1− w )/0.044 w ) in a single extraction step, but some come close. Hence, we retain the 64 structures with the highest P EtOH values and satisfying the additional constraint Q EtOH > Q water that emerge from this initial screening step for simulations at five higher w values that span the likely range of process conditions (0.43, 1.4, 4.5, 15 and 41 wt% selected from equilibrium raffinate concentrations observed in previous simulations for adsorption in MFI [9] ). Fortunately, as illustrated in Fig. 1 , S EtOH decreases at a slower rate than w increases for many zeolite structures. Thus, by raising w to 0.43 wt%, we find 18 structures capable of reaching a sufficiently high S EtOH to exceed the azeotropic point ( S target ≥5,100), and this number further increases for even larger raffinate concentrations. 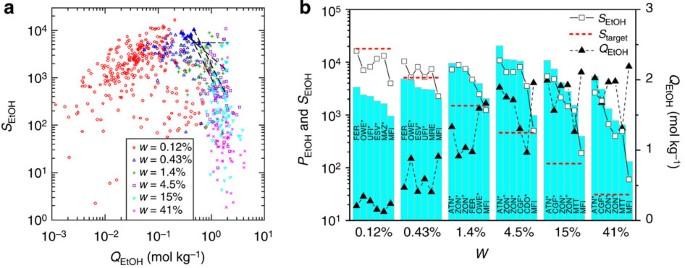Figure 1: Ethanol/water adsorption at different solution-phase concentrations. (a) Scatter plot of ethanol selectivity (SEtOH) versus loading (QEtOH). Filled symbols highlight the 10 highest ranked structures atw=0.43 and 15 wt% and dashed lines connect those structures found among the top 10 for bothw. (b) Adsorption characteristics (PEtOH=SEtOHQEtOH, cyan bars) for the top 5 zeolites (structure codes listed on bars) at eachw, with data for MFI shown for comparison. The horizontal red lines indicateStarget=0.956(1−w)/0.044w. Figure 1: Ethanol/water adsorption at different solution-phase concentrations. ( a ) Scatter plot of ethanol selectivity ( S EtOH ) versus loading ( Q EtOH ). Filled symbols highlight the 10 highest ranked structures at w =0.43 and 15 wt% and dashed lines connect those structures found among the top 10 for both w . ( b ) Adsorption characteristics ( P EtOH = S EtOH Q EtOH , cyan bars) for the top 5 zeolites (structure codes listed on bars) at each w , with data for MFI shown for comparison. The horizontal red lines indicate S target =0.956(1− w )/0.044 w . Full size image The adsorption characteristics of the top five framework types at all 6 w values are compared with MFI in Fig. 1b (numerical data for these high-performing zeolites are provided in Supplementary Table 1 ). FER is the top-ranked structure at w =0.12 and 0.43 wt% due to its exceptionally high S EtOH , and remains among the top 10 structures at w =1.4, 4.5 and 15 wt%. Its retentate exceeds the azeotropic composition for w ≥0.43 wt%. In contrast, MFI only exceeds S target for the three higher w and is not among the top 10 structures at any w . Three of the other top five structures (OWE*, ESV*, UFI*) currently exist only as aluminosilicates or aluminophosphates, whose adsorption properties may be different from the idealized siliceous structures (indicated by * added to the three-letter code) used for the screening. Nonetheless, the siliceous forms of these framework types will be attractive synthesis targets. As indicated in Fig. 1 , there is little correlation between selectivity and loading for w ≤1.4 wt%. Here, Q EtOH is very low in many cases and sufficient adsorption sites are present for both types of molecules. At w ≥4.5 wt%, one observes the typical compromise between selectivity and capacity: increasing w leads to increasing Q EtOH and decreasing S EtOH due to enhanced water co-adsorption. Selectivities at w =0.43% are a poor indicator of those at w =15% (with a correlation coefficient of R 2 =0.31), whereas S EtOH values at the two lowest and at the three highest concentrations are reasonably well correlated. This behaviour can be attributed to the fact that, for most frameworks, Q EtOH values at w =0.43 wt% are less than one-third of the values at w =15 wt%, whereas those at w =4.5 and 41 wt% are on average only ≈12% smaller and ≈5% larger than those at w =15 wt%; that is, these three raffinate concentrations fall into the flat part of the isotherm near saturation loading. For these highly non-ideal mixtures, the screening process must consider multiple feed concentrations and cannot simply rely on data at one w . Due to the differences in their adsorption characteristics, each material may have a different set of optimal operation conditions for a given process set-up. For example, FER may work best to extract 90% of the ethanol contained in a 5 wt% fermentation broth by an equilibrium-based adsorptive separation reaching down to a raffinate concentration of w =0.5 wt%. In contrast, ATN* continues to possess very high selectivity at much higher w . Therefore, processes using ATN* may choose to exploit the higher ethanol loadings at higher w , and reduce the feed mixture from an initial w of, say, 15 down to 5 wt% and recycle the raffinate back to the fermentation broth. Data at multiple w also allow us to find suitable combinations for a two-step separation utilizing two different zeolites. For example, structure VFI*, an aluminophosphate, reaches Q EtOH >2.0 mol kg −1 already at w =0.12 wt%, but with a relatively modest S EtOH =620. The retentate of this adsorption yields r =43 wt% and can be used as feed for another adsorption with ATN* that offers the highest S EtOH at w ≥4.5 wt%. Computation of the full adsorption isotherms and diffusivities would allow optimization of the operation conditions for single- or multi-step separations. Previous screening studies for simpler sorbates [11] , [13] have focused on finding structure–property relationships with the goal of identifying the geometric motifs responsible for the high performance of certain materials. However, the ethanol/water mixture exhibits significant non-idealities in both the solution and adsorbed phases due to strong intermolecular interactions [9] , and the common geometry–performance correlations do not appear to hold well for S EtOH , Q EtOH and P EtOH (see Supplementary Fig. 2 ). In Fig. 2 , we contrast the siting of the adsorbed molecules at w =0.43 wt% in FER with that in MFI, a zeolite heavily explored in the literature for its potential to separate ethanol from its aqueous solution [7] , [24] . In MFI, the enlarged intersection regions of the two channel systems facilitate water molecules with multiple hydrogen bonds, which reduces the energetic penalty for transferring water from its bulk environment and lowers the selectivity for ethanol. On the other hand, the distribution of adsorption sites in FER is such that two adjacent favourable sites for ethanol are spaced far enough apart that an extended hydrogen-bonding network involving water is not formed. At w =15 wt%, ethanol populates the other FER channels that permit some hydrogen bonding and S EtOH decreases twofold. As seen in Fig. 2 , the high Q EtOH and modest S EtOH in VFI* are due to 1.2-nm channels that are less hydrophobic than smaller channels and allow for significant loading ( Q water > Q EtOH ) even at w =0.12 wt%, whereas the high S EtOH in ATN* at high w =15 wt% is caused by well-spaced ethanol adsorption sites separated by narrow windows. The inherent complexity of these specific cases is not captured by the more commonly used geometric parameters, and much more complex combinations of geometric factors are needed to capture the performance at different raffinate concentrations. 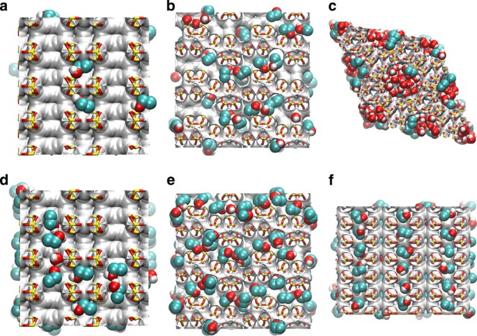Figure 2: Snapshots of representative ethanol/water configurations inside zeolite frameworks. (a) FER atw=0.43 wt%, (b) MFI at 0.43 wt%, (c) VFI* at 0.12 wt%, (d) FER atw=15 wt%, (e) MFI atw=15 wt% and (f) ATN* atw=15 wt%. Silicon, oxygen, carbon and hydrogen atoms are shown as yellow, red, cyan and white, respectively. Isosurfaces equidistant to framework atoms are shown in grey. Figure 2: Snapshots of representative ethanol/water configurations inside zeolite frameworks. ( a ) FER at w =0.43 wt%, ( b ) MFI at 0.43 wt%, ( c ) VFI* at 0.12 wt%, ( d ) FER at w =15 wt%, ( e ) MFI at w =15 wt% and ( f ) ATN* at w =15 wt%. Silicon, oxygen, carbon and hydrogen atoms are shown as yellow, red, cyan and white, respectively. Isosurfaces equidistant to framework atoms are shown in grey. Full size image Separation of long-chain hydrocarbons Hydroisomerization is a modern dewaxing technique that uses certain zeolites as bifunctional catalysts with incorporated group VIII metals to selectively convert ‘waxy’ linear long-chain alkanes to their ‘less waxy’ slightly branched isomers possessing a high viscosity index, without much cracking into less valuable low-molecular-weight alkanes. The framework structures of the high-performing zeolites for this application can promote the adsorption of linear alkanes and have high separation factors over branched alkanes. Adsorption using the siliceous forms of the same zeolite framework types are also desired in, for example, the UOP Molex process [1] for separating the branched alkanes used in transportation fuels from the linear ones used to produce plasticizers and synthetic detergents. Previously, Dubbeldam et al . [25] screened about 100 nanoporous materials for the adsorption of hexane and heptane isomers. We here screen >330,000 zeolite structures in the IZA-SC and PCOD databases [10] , [23] . To represent the complex hydrocarbon feed, we use an equimolar mixture of n -octadecane (C18), n -tetracosane (C24), n -triacontane (C30), 2-methyl and 4-methylheptadecane (2C17 and 4C17), and 2,2-dimethylhexadecane (22C16). Three indicators are constructed to characterize performance: (i) high affinity towards linear alkanes so that they will be present at high concentrations near the active sites within the framework, as indicated by Henry's constant, k H,C18 , at the infinite-dilution limit or loading, Q C18 , at P =3 MPa for C18; (ii) high selectivity for linear-versus-branched alkanes so that the branched products, once formed, will be quickly desorbed to prevent further cracking, as indicated by S B p =3 y C18 /( y 2C17 + y 4C17 + y 22C16 ) where p =0 (the infinite-dilution limit) or 3 MPa and y = k H or Q depending on state point; and (iii) low selectivity between linear alkanes of different lengths as indicated by S L p =( y C24 y C30 ) 1/2 / y C18 so that a broad range of linear alkanes will be converted; the resulting performance metric is P HC p = y C18 S B p / S L p . The first screening step aims to reduce the number of candidate materials using relatively short simulations performed at T =573 K and the infinite-dilution limit. Screening the IZA-SC database [23] reveals that six of the top seven structures (ATO, MRE, MTT, AFO, MTW and FER) are already described in patents for isodewaxing [2] , [3] and the primary literature [4] , [5] . This strongly indicates that our screening procedure, although based solely on adsorption properties, is able to capture the essential characteristics responsible for high-performing hydroisomerization catalysts and can thus provide useful guidance for experimental synthesis of novel zeolite catalysts. Thus, we expand the pool of candidate materials to include zeolite-like structures in the PCOD database [10] . Due to the weak correlation between data at the infinite-dilution limit and at finite pressure for some of the performance indicators (see below), materials that are among the top 64 in the IZA-SC database or top 1,024 in the PCOD database in any of the three performance indicators (for a total of 103 and 2,835 structures, respectively) are retained for longer simulations in the infinite-dilution limit and for the same equimolar mixture at T =573 K and p =3 MPa, a typical operation condition for the hydroisomerization process [1] . 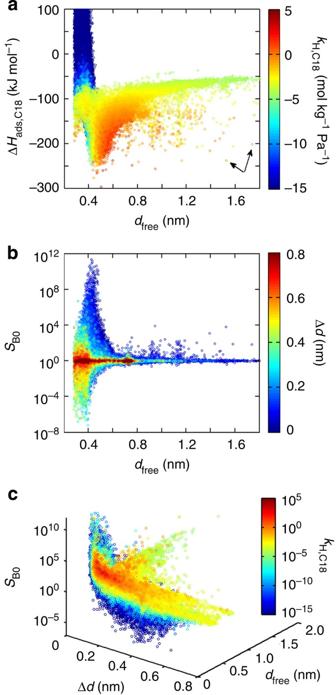Figure 3: Hydrocarbon adsorption at the infinite-dilution limit for all IZA-SC and PCOD structures. (a) Scatter plot of the adsorption enthalpy for C18 (ΔHads,C18) versus the free pore diameter (dfree) with the colour scheme indicating Henry’s constant (kH,C18). (b) Scatter plot of linear-versus-branched selectivity (SB0) versusdfreewith the colour scheme indicating the pore bumpiness (Δd). (c) Scatter plot ofSB0versus Δdanddfreewith the colour scheme indicatingkH,C18. Figure 3a illustrates the relationships between k H,C18 , the adsorption enthalpy, Δ H ads,C18 , and the free channel diameter, d free , given by the diameter of the largest sphere that can roam freely through the channel [26] , for C18 adsorption in the infinite-dilution limit. A more favourable Δ H ads,C18 generally leads to a larger k H,C18 , but the correlation is fairly weak. This reflects enthalpy–entropy compensation where a smaller entropic loss in a somewhat wider channel can compensate for a smaller enthalpic gain, as seen by the cloud of data points with the largest k H,C18 values (shown in red and orange in Fig. 3a ). The majority of these zeolites with favourable adsorption characteristics are found for 0.45 nm< d free <0.75 nm, but there is a significant number of outliers particularly at large d free values. These outliers are associated with zeolites containing multiple channels, where the channel with the largest d free makes only a negligible contribution to the adsorption characteristics at the infinite-dilution limit. Two of these structures are highlighted by arrows in Fig. 3a . The zeolite structure with d free =1.74 nm contains another channel with d free =0.59 nm, and that with d free =1.53 nm contains two other channels with d free =0.50 and 0.29 nm. For the latter example, it is the intermediate channel that governs the adsorption characteristics at the infinite-dilution limit; that is, using the d free values of the smallest channel would also lead to many outliers. The very large spread of Δ H ads,C18 and k H,C18 values for d free <0.45 nm can be attributed to the fact that neither the overall shape nor the cross-section of the C18–C30 alkanes is well described by a sphere or a circle, respectively, in contrast to simpler molecules (for example, methane with fairly spherical shape and carbon dioxide and nitrogen with fairly circular cross-sections). For the alkanes, a better geometric descriptor for the cross-section would certainly be an ellipse, but this can only be described by two parameters. Zeolite structures with d free <0.45 nm and favourable adsorption characteristics possess channels with larger differences between the minor and major elliptical axis, whereas those with unfavourable adsorption characteristics are more circular in cross-section. These geometric descriptors also do not account for the arrangement of framework atoms away from the pore surface that contribute to a favourable Δ H ads . This discussion illustrates the need for detailed computation in addition to geometric rules of thumb to evaluate adsorption performance for complex sorbates. Figure 3: Hydrocarbon adsorption at the infinite-dilution limit for all IZA-SC and PCOD structures. ( a ) Scatter plot of the adsorption enthalpy for C18 (Δ H ads,C18 ) versus the free pore diameter ( d free ) with the colour scheme indicating Henry’s constant ( k H,C18 ). ( b ) Scatter plot of linear-versus-branched selectivity ( S B0 ) versus d free with the colour scheme indicating the pore bumpiness (Δ d ). ( c ) Scatter plot of S B0 versus Δ d and d free with the colour scheme indicating k H,C18 . Full size image A strong affinity for C18, as indicated by large k H,C18 values, is well correlated with an even stronger affinity for C24 and C30, that is, large S L0 , but not correlated with a preference for linear-versus-branched alkanes, that is, large S B0 . We find that S B0 is best correlated with the pore bumpiness, Δ d =Δ d incl − d free , where the first term is the diameter of the largest sphere that can be placed anywhere along a given channel [26] . As shown in Fig. 3b , high selectivity for linear alkanes is usually associated with a narrow ( d free <0.45 nm) and smooth channel (Δ d <0.1 nm), whereas inverse selectivity, which prefers adsorption of the branched alkanes, tends to occur for even narrower ( d free <0.4 nm) but bumpy channels with Δ d ≈0.3 nm. Most of the structures with large inverse selectivity also exhibit very low affinity for any alkane as indicated by k H,C18 / S B0 <10 −5 (see Fig. 3c ). In general, zeolite structures with d free >0.6 nm and/or Δ d >0.6 nm are not selective for the different alkane isomers. The outliers found for larger d free values are again due to zeolite structures with multiple channels, where the selectivity for linear alkanes is associated with a smaller channel. It is noteworthy that the spread of these geometry–property correlations is again fairly large, limiting the utility of using simple geometric descriptors to predict adsorption properties of complex, articulated molecules. 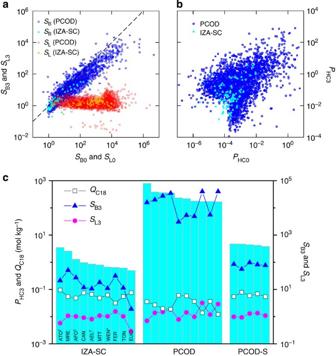Figure 4: Hydrocarbon adsorption at high pressure. Scatter plots of (a) linear-versus-branched (SBp) and long-versus-short (SLp) selectivities and of (b) performance score (PHCp) atp=3 MPa versus those in the infinite-dilution limit for all structures retained after the first screening step. (c) Adsorption characteristics (PHC3=QC18SB3/SL3, bars) for the top 10 IZA-SC and PCOD structures and for PCOD-S structures with similar selectivities as the IZA-SC structures. The seven-digit PCOD structure identifiers are given inSupplementary Table 2. Figure 4a,b compare adsorption characteristics calculated in the infinite-dilution limit and at hydroisomerization conditions. For both IZA-SC and PCOD structures, the two selectivities exhibit markedly different trends as pressure is increased: S B values are fairly insensitive to pressure changes and, hence, well correlated, whereas S L diminishes for the majority of zeolites as pressure increases. Longer alkanes have much smaller vapour pressures and, correspondingly, the free energy penalty for them to leave the liquid phase is larger than for shorter alkanes and compensates for the more favourable free energy of adsorption. As a result, S L reduces to around 1–10 at p =3 MPa. As expected, there is only a weak correlation between the infinite-dilution affinity and the high pressure loading (see Supplementary Fig. 3 ) because larger pores allow for higher loading but are not most favourable for individual sorbates. For the combined performance score, P HC , a modest correlation is observed between the two conditions. The complex pressure dependencies illustrate the shortcomings of using infinite-dilution data to extrapolate material performance at other conditions and are the reason to retain structures performing well in any of the three performance indicators and not just those with the highest performance score for the next screening step. Figure 4: Hydrocarbon adsorption at high pressure. Scatter plots of ( a ) linear-versus-branched ( S B p ) and long-versus-short ( S L p ) selectivities and of ( b ) performance score ( P HC p ) at p =3 MPa versus those in the infinite-dilution limit for all structures retained after the first screening step. ( c ) Adsorption characteristics ( P HC3 = Q C18 S B3 / S L3 , bars) for the top 10 IZA-SC and PCOD structures and for PCOD-S structures with similar selectivities as the IZA-SC structures. The seven-digit PCOD structure identifiers are given in Supplementary Table 2 . Full size image Figure 4c compares the top 10 structures (as ranked by P HC3 ) from each database (numerical values are provided in Supplementary Table 2 ). The top 3 (ATO, MRE and AFO) and another four (AEL, MTT, FER and TON) from the top 10 IZA-SC structures are known to excel for this petrochemical application [2] , [3] , [4] , [5] ; fourth and seventh ranked CAN and WEN* have performance indicators resembling the other structures, whereas tenth ranked EUO yields a lower S B3 that is compensated by a more favourable S L3 . Top-ranked ATO features the highest Q C18 , the second lowest (favourable) S L3 , and the fourth highest S B3 . The largest variation among the top 10 IZA-SC structures is found for S B3 that range from 2–50, whereas the smallest and largest values of Q C18 and S L3 vary only by factors of 3 and 5. The top 10 PCOD structures exhibit P HC3 values that are about two orders of magnitude higher than those for the high-performing IZA-SC structures. This dramatically improved performance arises mainly from their exceptionally high S B3 values, whereas their Q C18 and S L3 values tend to be slightly less favourable than for the IZA-SC structures. As indicated by the five structures labelled PCOD-S, this database contains also structures that match the Q C18 and S L3 values of the top IZA-SC performers and still outperform them. The performance differences are much larger in the infinite-dilution limit where some PCOD structures yield k H,C18 and S B0 values that exceed those of the IZA-SC structures by 3 and 7 orders of magnitude, respectively (see Supplementary Table 2 and Supplementary Fig. 4 ). In Fig. 5 , we compare the arrangement of the adsorbed hydrocarbons in ATO, MTW and PCOD-8113534. As can be seen, the top-performing structures all possess one-dimensional 12-ring channel architectures and these systems are near saturation loading at P =3 MPa. ATO and PCOD-8113534 are the top-ranked IZA-SC and PCOD structures and also perform exceptionally well at the infinite-dilution limit. MTW is a patented framework type and is the sixth-ranked structure at infinite dilution, but only ranks 28th at P =3 MPa because of a large decrease in S B . The S B3 values for these three structures are 21, 2.8 and 16,000, respectively. As expected from the large S B3 , in the elliptical channels of PCOD-8113534 with a semiminor axis length of only 0.47 nm, the linear alkanes are highly confined with a preference to have their zig-zag plane aligned along the semimajor elliptic axis and exhibit very few gauche defects at the chain termini. ATO’s channels possess a cross-section resembling a regular hexagon with d free =0.57 nm, and the zig-zag plane of the alkanes is free to rotate; in addition to end-gauche defects, kink defects ( gtg ′) are also observed. The even larger elliptical channels in MTW afford sufficient room for few 22C16 molecules and gttg ′ kinks in linear chains. Herm et al . [27] recently investigated the separation of hexane isomers and found extremely high selectivity in a metal–organic framework with one-dimensional channels and a triangular cross-section. In the latter work, however, the desired selectivity to improve gasoline quality is for linear and mono-branched alkanes versus di-branched alkanes, whereas the desired selectivity is for linear versus mono- and di-branched alkanes in the present study. 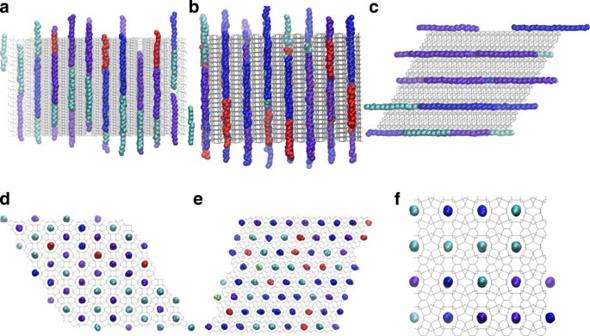Figure 5: Snapshots of representative hydrocarbon configurations inside zeolite frameworks. The adsorption occurs from a liquid phase containing an equimolar hydrocarbon mixture atT=573 K andP=3 MPa. Views facing the main channel axis (a–c) and along the main channel axis (d–f) are shown for ATO (a,d), MTW (b,e) and PCOD-8113534 (c,f). Zeolite frameworks are depicted as grey lines, and C18, C24, C30, (2C17 and 4C17) and 22C16 molecules as cyan, purple, blue, red and green spheres, respectively. Figure 5: Snapshots of representative hydrocarbon configurations inside zeolite frameworks. The adsorption occurs from a liquid phase containing an equimolar hydrocarbon mixture at T =573 K and P =3 MPa. Views facing the main channel axis ( a – c ) and along the main channel axis ( d – f ) are shown for ATO ( a , d ), MTW ( b , e ) and PCOD-8113534 ( c , f ). Zeolite frameworks are depicted as grey lines, and C18, C24, C30, (2C17 and 4C17) and 22C16 molecules as cyan, purple, blue, red and green spheres, respectively. Full size image The type of materials discovery presented here focuses on core characteristics of a technology, such as the ethanol selectivity and capacity for ethanol/water separation and the adsorption affinity for linear alkanes and two different selectivities concerning carbon chain length and degree of branching for hydroisomerization dewaxing. The performance metrics chosen in this work are not tied to any specific process, but aim to identify optimal materials that will likely perform well in a range of processes. The best operation modes and process conditions may be different for each material and feedstock composition, and the ranking may vary once a particular process is selected [28] , [29] . In addition, practical considerations will sometimes dictate the suitability of a process. For example, solids contained in the fermentation broths can plug the porous sorbent and prevent the use of separation processes involving direct contact with the solution phase. Other factors related to, say, economics and logistics, will also impact the attractiveness or even feasibility of using a particular material in an actual plant. The materials performance data obtained here are hence best viewed as a starting point on the technology readiness ladder. As is common in any application of computer-aided engineering concepts, significant challenges exist between the design phase and the practical application. The experimental discovery of new zeolites usually takes a long time, lots of skill and some luck. Additional hurdles need to be surmounted to synthesize nearly defect-free, all-silica materials that are beneficial for the ethanol/water separation or to embed the catalytic sites needed for the hydroisomerization reaction. Significant advances in this area will be required before it becomes feasible to systematically synthesize and test predicted zeolite structures or defect-free, all-silica variants of already-known zeolite frameworks. Some candidate zeolite structures that are thermodynamically feasible may prove to be synthetically inaccessible due to kinetic barriers in the crystallization process [30] . Recently, Schmidt et al . [31] succeeded in using computationally predicted organic structure directing agents to synthesize a particular, specified zeolite; an important step in the synthesis of tailor-made zeolites. In light of these obstacles, being able to narrow down the list of potentially attractive synthesis targets becomes even more crucial. In related work, Gomez-Gualdron et al . [32] reported on the synthesis and measured storage capacity of a metal–organic framework that was computationally predicted to be a promising material due to alkyne groups being placed close to the metal nodes. In conclusion, this work displays the benefits provided by computational screening for increasing the speed of materials discovery. Enabled by advanced algorithms, accurate intermolecular potentials, and massively parallel computer architectures, we are now able to expedite hundreds of thousands of virtual experiments for complicated systems of industrial relevance. Data mining using differently tuned objective functions affords the opportunity to adapt to process conditions or desired products. Framework structures The IZA-SC database [23] used in our screening consists of a set of idealized framework structures and other experimentally determined structures. The idealized structure for each framework type is obtained by geometric refinement with prescribed interatomic distances, assuming a (hypothetical) SiO 2 composition, and in the highest possible symmetry space group of the framework type. The experimental structures are included for the screening if they contain only O, Si, Al, P or H atoms after removal of any solvent molecules and ions and resolution of partial occupation numbers by proportional random assignments on the unit cell level, followed by replacement of Al and P atoms with Si atoms. Together, the idealized and experimental IZA-SC structures yield 402 unique sorbents. The larger PCOD database [10] was constructed by enumerating space groups, unit cells, density and sampling coordinates of Si atoms in the irreducible unit. The resulting 2.6 million candidate structures were geometry optimized and, based on an energetic criterion, 331,172 structures are considered as thermodynamically accessible [10] . A performance rank is given here only to structures that have accessible pores/channels [26] . Force fields The transferable potentials for phase equilibria (TraPPE) and TIP4P force fields are used to model zeolites [33] , hydrocarbons [34] , [35] , ethanol [36] and water [37] . The TraPPE-zeo force field for all-silica zeolites [33] treats dispersive and first-order electrostatic interactions in a balanced manner and, hence, allows one to study a wide range of sorbate molecules. The combination of TraPPE-zeo and the sorbate models has been extensively validated in systems closely related to the two applications reported in this work, including the adsorption and diffusion of alkanes, CO 2 , alcohols and H 2 O in different zeolite structures, across a wide range of temperatures and pressures [33] , [38] , [39] . All sorbate–sorbate interactions are evaluated explicitly to a cut-off distance of 1.4 nm, while the long-range Lennard-Jones (LJ) contributions are estimated via tail corrections and the first-order electrostatics are treated with the Ewald summation technique [40] . In our simulations, the zeolite frameworks are assumed to be rigid, while sorbate molecules sample angle bending and dihedral motions. To improve computational efficiency, grid files for the interaction energy of a test particle with the zeolite [41] are generated in a manner that contains the repulsive and the attractive LJ (including the contribution from the tail corrections), and the direct-space and reciprocal-space Coulomb components, but is independent of the specific force-field parameters for the sorbate molecule; therefore the same grid files can facilitate screening calculations for other applications. Simulation methods Configurational-bias Monte Carlo simulations in the grand-canonical ensemble (CB-GCMC) [40] , [42] are used to compute sorbate loadings as a function of either the concentration of the ethanol/water bulk solutions or partial pressures for the hydrocarbon mixtures. The chemical potentials required for these simulations are obtained from previous Gibbs ensemble simulations with explicit solution phases [9] (hence, the specific choices of raffinate concentrations used here) or determined from liquid-phase simulations in the isobaric–isothermal ensemble for the alkanes. The coupled–decoupled configurational-bias Monte Carlo (CD-CBMC) algorithm [35] is used to enhance the sampling of intramolecular degrees of freedom and to improve the acceptance rates of GCMC insertion/deletion moves. In addition, CD-CBMC identity switch moves [43] , which convert between different hydrocarbon molecules, are used to further assist the sampling of the sorption equilibria. In the infinite-dilution limit where sorbate–sorbate interactions are negligible (realized by setting the chemical potentials to very negative values so that insertion moves are never accepted), these CB-GCMC simulations also yield directly k H and Δ H ads (ref. 42 ). To carry out the energy grid tabulation and CB-GCMC simulations in a high-throughput fashion, we implement a two-level parallel execution hierarchy exploring simultaneously 2 7 to 2 14 zeolite structures and accelerating the simulations for each structure by spreading the computational load over 2 2 to 2 8 compute cores. For the ethanol/water adsorption isotherm, 10 6 MC steps were performed at each concentration. For the hydrocarbon dewaxing application, 9 × 10 4 MC steps were used for the initial screening at infinite dilution, and a total of 9 × 10 5 and 1.6 × 10 6 MC steps were performed for the top structures to obtain better statistics for the infinite-dilution properties and to compute the liquid-mixture properties, respectively. These massively parallel screening calculations were performed on Mira, a leadership-class supercomputer at Argonne National Laboratory. Screening workflow For the ethanol/water separation, a two-step screening workflow is utilized where the adsorption properties are computed for all 402 idealized and experimental IZA-SC structures at only the lowest solution-phase concentration ( w =0.12 wt%). The 64 structures with the highest P EtOH values and satisfying the additional constraint Q EtOH > Q water that emerge from this initial screening step are retained for the second step that involves simulations at five higher concentrations. For the hydrocarbon dewaxing application, the first screening step involves the calculation of the Henry’s constants for the six hydrocarbons and the corresponding selectivities from relatively short simulations in all 402 IZA-SC and 331,172 PCOD structures. On the basis of being among the 64 or 1,024 top-performing structures in the IZA-SC or PCOD databases, respectively, in any of the three performance indicators (largest k H,C18 , largest S B0 , and smallest S L0 ), 103 IZA-SC and 2,835 PCOD structures are retained for the second step that involves longer simulations probing adsorption in the infinite-dilution limit and from the solution phase. The performance indicators obtained from the short and long simulations at the infinite-dilution limit are highly correlated for the PCOD structures with correlation coefficients ranging from 0.79 to 0.97 and support retaining only ≈1% of the structures (see Supplementary Fig. 5 ). The correlation coefficient for S B0 obtained for the IZA-SC structures is only 0.31, but values of 0.73 and 0.97 are found for S L0 and k H,C18 , respectively. In this case, ~30% of the structures are retained for the second step. Validation experiments To validate the predictions for the ethanol/water separation, solution-phase adsorption isotherms are measured in high-quality samples of MFI (silicalite-1) and FER (ferrierite). The ethanol loading in MFI and FER predicted using the current simulation protocol and measured experimentally are compared in Fig. 6 , and the predictions agree very well with the experimental data. It should be noted that decreasing the presence of defects or increasing the temperature shifts the ethanol adsorption isotherm to higher concentrations/lower loadings. (Additional validation data related to ethanol/water separation is provided in Supplementary Fig. 6 .) The preparation procedure for MFI [44] and FER [45] are as follows. The MFI samples are prepared from starting molar composition of 1.0 SiO 2 :0.08 TPABr:0.4 NH 4 F:20 H 2 O where 1.66 g of tetrapropylammonium bromide (98%, Aldrich) is added to 27.62 g of distilled water followed by the addition of 1.15 g of ammonium fluoride (98%, J.T. Baker). After vigorously stirring at room temperature for 15 min, 4.61 g of silica (SiO 2 , Cabosil M5, Riedel de Haën) is added and then the whole solution is hand-mixed with a spatula until the solution appeared homogeneous. The mixture is transferred into a Teflon-lined stainless-steel autoclave and thermally treated at 448 K for 7 days in static condition. The resulting MFI crystals are washed by repeated centrifugation at a relative centrifugal force of 20,000 for 20 min until the supernatant pH is neutral. The solid from centrifugation is dried in a convection oven at 343 K overnight. The dried MFI crystals are calcined at 823 K at a ramp rate of 1 K min −1 for 20 h under 100 ml min −1 of dry air flow and subsequently cooled to room temperature. The FER samples are prepared from starting molar composition of 1.5 SiO 2 :2.0 HF/Pyr:4 H 2 O:8 PrNH 2 :16 Pyr where 1.05 g of HF/Pyr (Hydrogen fluoride pyridine, HF:Pyr ≈70:30, Aldrich) is added to 23.3 g of pyridine (98%, Aldrich) followed by the addition of 8.7 g of PrNH 2 ( n -Propylamine, 98%, Aldrich) and 1.32 g of distilled water. After stirring at room temperature for 45 min, 1.66 g of silica (SiO 2 , Cabosil M5, Riedel de Haën) is added to the clear solution under vigorous stirring. The final gel is formed after 2 h mixing. The mixture is transferred to a Teflon-lined stainless steel autoclave and thermally treated in an oven at 453 K for 7–10 days in static condition. The dried FER is calcined at 1123 K at a ramp rate of 1 K min −1 for 16 h under 100 ml min −1 of oxygen flow and subsequently cooled to room temperature. For the adsorption measurements [44] , ethanol (200 proof, Fisher Scientific) is diluted with distilled water to prepare concentrations ranging from 0.05 to 5 wt% of ethanol solution. 0.4 ml of the ethanol solution is transferred into a closed glass vial and subsequently from 50 mg to 180 mg of zeolite adsorbent is added. The zeolite-solution mixture is stirred until equilibration in a water bath where the temperature is controlled at 298±0.5 K. Each solution is filtered with a 1 ml Monojet syringe connected to a 0.2 μm GHP (polypropylene) syringe filter to remove the zeolite particles. The filtrate concentration is analysed by using an Agilent 1200 High Performance Liquid Chromatography equipped with a refractive index detector (RID) and an autosampler. The autosampler injects a 20 μl sample into a stream of 0.005 M sulfuric acid (H 2 SO 4 ) with a flow rate of 0.5 ml min −1 . The stream is passed through a Bio-Rad Aminex HPX-87H polystyrene-packed column heated to 333 K. The outlet stream is passed through a RID, which is heated to 323 K and the RID signal is recorded and plotted with respect to time. The relative signal intensities of the ethanol and a glycerol (99.5%, Aldrich) internal standard are used to estimate the final concentration of each solution. The difference between the initial and final concentration of ethanol and the total volume of the solution is used to determine the adsorbed ethanol amount, but the measurement is not sensitive enough to quantify the amount of water. 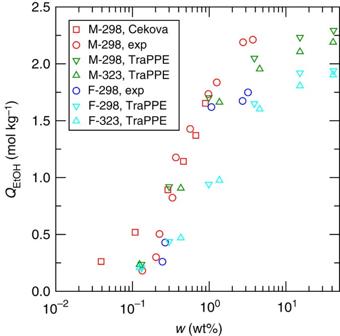Figure 6: Comparison of adsorption isotherms for ethanol/water solutions. The red squares, red circles and blue circles show the experimental data atT=298 K in MFI measured by Cekovaet al.46, and in MFI and FER, respectively, from the validation experiments carried out as part of this study. The predictions using the TraPPE-zeo/TraPPE-UA/TIP4P force fields are shown as green down and up triangles for MFI atT=298 and 323 K, respectively, and as cyan down and up triangles for FER at 298 and 323 K, respectively. Figure 6: Comparison of adsorption isotherms for ethanol/water solutions. The red squares, red circles and blue circles show the experimental data at T =298 K in MFI measured by Cekova et al . [46] , and in MFI and FER, respectively, from the validation experiments carried out as part of this study. The predictions using the TraPPE-zeo/TraPPE-UA/TIP4P force fields are shown as green down and up triangles for MFI at T =298 and 323 K, respectively, and as cyan down and up triangles for FER at 298 and 323 K, respectively. Full size image How to cite this article: Bai, P. et al . Discovery of optimal zeolites for challenging separations and chemical transformations using predictive materials modeling. Nat. Commun. 6:5912 doi: 10.1038/ncomms6912 (2015).